Mechanism for full-length RNA processing ofArabidopsisgenes containing intragenic heterochromatin Genomes of higher eukaryotes contain many transposable elements, which often localize within the transcribed regions of active genes. Although intragenic transposable elements can be silenced to form heterochromatin, the impact of intragenic heterochromatin on transcription and RNA processing remains largely unexplored. Here we show using a flowering plant, Arabidopsis , that full-length transcript formation over intragenic heterochromatin depends on a protein named IBM2 (Increase in Bonsai Methylation 2), which has a Bromo-Adjacent Homology domain and an RNA recognition motif. Mutation of ibm2 triggers premature termination of transcripts with 3′ RNA processing around intragenic heterochromatin at loci including the H3K9 demethylase gene IBM1 . The need for IBM2 is circumvented in variant alleles that lack the heterochromatic domain. Our results reveal a mechanism that masks deleterious effects of intragenic heterochromatin, providing evolutionary sources for genetic and epigenetic variations. Genomes of vertebrates and plants contain a substantial number of transposable elements (TEs) [1] , which are silenced by repressive epigenetic modifications, such as cytosine methylation and methylation of lysine 9 of histone H3 (H3K9me) [2] . These modifications are essential for the formation of inactive chromatin structures called heterochromatin. In contrast, these modifications are generally excluded from active genes, which depend on passage of the transcription machinery [3] , [4] , [5] . A potential complication is that active cellular genes sometimes contain TEs within their transcribed regions, particularly in higher eukaryotes with large genomes [6] , [7] , [8] . Intragenic TEs can cause modulation of gene expression, truncation of transcripts, and creation of poly(A) sites and alternative splicing sites [9] . In mammals, for example, the intragenic intra-cisternal A particle (IAP) retrotransposon triggers premature termination of transcripts at cryptic poly(A) signals within or even outside the element, depending on differential DNA methylation of the element [10] , [11] . In plants, heterochromatic epigenetic modifications at TEs are established by RNA interference (RNAi)-mediated mechanisms called RNA-directed DNA methylation, and are maintained by DNA methylases and by chromatin remodelling factor [2] , [12] . In general, TEs associated with heterochromatin accumulate at pericentromeric regions of chromosomes [13] , [14] , whereas a substantial number of TEs are also found within gene units, particularly in introns [8] , [15] , [16] . Despite their abundance, however, epigenetic regulation of intragenic TEs and their impact on modes of transcription remain largely unexplored. In this study we show that heterochromatic epigenetic modifications are commonly found within actively transcribed gene units in both the Arabidopsis and rice genomes. We further show that in Arabidopsis , full-length transcription of genes with intragenic heterochromatin, most of which is formed by TE insertions, requires IBM2 (Increase in Bonsai Methylation 2), a protein with a Bromo-Adjacent Homology (BAH) domain and an RNA recognition motif (RRM). Our results reveal an epigenetic mechanism that masks the effects of genetic variations created by TE insertions, allowing evolution of complex genomes with heterochromatic domains having diverse functions. IBM2 controls full-length transcription of IBM1 locus In the flowering plant, Arabidopsis , H3K9 methylation and DNA methylation are generally excluded from genic regions by the action of H3K9 demethylase IBM1 (refs 17 , 18 , 19 ). ibm1 mutants show developmental defects and ectopic accumulation of H3K9me and DNA methylation at non-CG sites, for thousands of transcribed genes [17] , [18] , [19] . In the course of this study, we identified a novel factor named IBM2 that is required for proper expression of IBM1 . A mutant of IBM2 ( AT5G11470 ) was isolated from a genetic screen as ibm1 ; however, the gene encodes a previously uncharacterized protein that has a BAH domain near the N terminus and an RRM in the C-terminal part ( Fig. 1a , Supplementary Fig. S1a ). ibm2 mutants show phenotypes very similar to those of ibm1 mutants. In both mutants, non-CG DNA methylation accumulated in genic regions ( Supplementary Figs S1–S3 ), whereas repeat sequences were unaffected ( Supplementary Fig. S4 ). Ectopic genic non-CG methylation and developmental defects in the mutants depend on the functions of both histone H3K9 methylase KRYPTONITE (KYP) and DNA methylase CHROMOMETHYLASE3 (CMT3; Supplementary Fig. S5 ). These observations suggest that IBM2 acts on the same genetic pathway as IBM1 ( Supplementary Fig. S6 ). 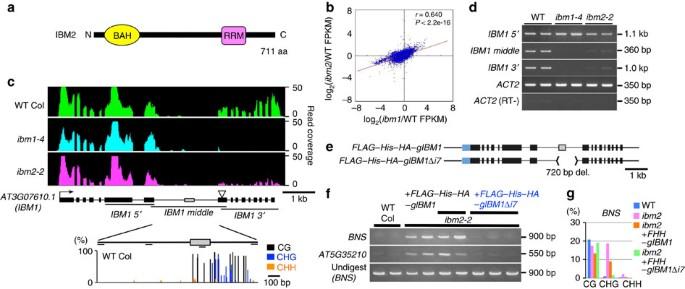Figure 1: IBM2 regulates transcription ofIBM1. (a) A schematic representation of the IBM2 protein. BAH, Bromo-adjacent homology domain; RRM, RNA recognition motif. (b) A comparison of expression profiles betweenibm1andibm2by mRNA-seq. Each dot represents genes (n=18,920). Pearson’srandP-value (two-tailedt-test) are indicated. FPKM, Fragments per kilobase of transcript per million fragments mapped. (c) Top panel: Read coverage of theIBM1transcript in each genotype. Middle: Structure of theIBM1locus. Exons ofIBM1and insertion of the organelle genome are shown by black and grey boxes, respectively. The T-DNA insertion site of theibm1-4allele is shown with a white triangle. Bottom: Bisulphite analysis of the seventh intron ofIBM1in wild-type Columbia (Col). (d) RT–PCR ofIBM1transcripts from the regions indicated incdetected by 28–30 cycles of PCR. Each lane represents independent biological replication with the indicated genotypes. (e)IBM1transgenes used for complementation ofibm2-2mutant. Blue boxes represent FLAG–His–HA tags. (f) DNA methylation analysis ofBNSandAT5G35210detected by methylation-sensitive restriction digestion usingBglII followed by PCR.FLAG–His–HA-gIBM1Δi7rescued theibm2phenotypes. However,FLAG–His–HA–gIBM1with the heterochromatin region did not rescueibm2phenotypes. Each lane represents DNA methylation of independent transgenic plants (T1) with the indicated transgene. (g) The percentage of methylated cytosines atBNSin the plants examined inf. Figure 1: IBM2 regulates transcription of IBM1 . ( a ) A schematic representation of the IBM2 protein. BAH, Bromo-adjacent homology domain; RRM, RNA recognition motif. ( b ) A comparison of expression profiles between ibm1 and ibm2 by mRNA-seq. Each dot represents genes ( n =18,920). Pearson’s r and P -value (two-tailed t -test) are indicated. FPKM, Fragments per kilobase of transcript per million fragments mapped. ( c ) Top panel: Read coverage of the IBM1 transcript in each genotype. Middle: Structure of the IBM1 locus. Exons of IBM1 and insertion of the organelle genome are shown by black and grey boxes, respectively. The T-DNA insertion site of the ibm1-4 allele is shown with a white triangle. Bottom: Bisulphite analysis of the seventh intron of IBM1 in wild-type Columbia (Col). ( d ) RT–PCR of IBM1 transcripts from the regions indicated in c detected by 28–30 cycles of PCR. Each lane represents independent biological replication with the indicated genotypes. ( e ) IBM1 transgenes used for complementation of ibm2-2 mutant. Blue boxes represent FLAG–His–HA tags. ( f ) DNA methylation analysis of BNS and AT5G35210 detected by methylation-sensitive restriction digestion using Bgl II followed by PCR. FLAG–His–HA-gIBM1 Δ i7 rescued the ibm2 phenotypes. However, FLAG–His–HA–gIBM1 with the heterochromatin region did not rescue ibm2 phenotypes. Each lane represents DNA methylation of independent transgenic plants (T1) with the indicated transgene. ( g ) The percentage of methylated cytosines at BNS in the plants examined in f . Full size image Expression profiles of wild-type Columbia (Col), and ibm1 and ibm2 mutants were investigated by mRNA-seq analysis ( Supplementary Table S1 ). Target genes of IBM1 and IBM2 largely overlap, and overall expression changes showed a moderate correlation between ibm1 and ibm2 mutants (Pearson’s r =0.640, P <2.2e–16: Fig. 1b , Supplementary Fig. S7 ). Most importantly, the ibm2 mutant showed a significant reduction of IBM1 transcription at the 3′ region ( P =5.2e–21, Fisher’s exact test: Fig. 1c , Supplementary Data 1 ), which could account for the observed ibm1 -like phenotypes in the ibm2 mutant. The reduction of IBM1 transcript levels at the 3′ region occurred downstream of the seventh intron of IBM1 . This intron contains a 200-bp DNA fragment insertion that is homologous to part of ycf1 , encoded by both chloroplast and mitochondrial genomes ( Fig. 1c ). Bisulphite sequence analysis and database searches revealed that the ycf-like sequence is marked by DNA methylation at both CG and non-CG sites, and associated with small RNA production, generating a constitutive heterochromatic domain longer than 700 bp ( Fig. 1c , Supplementary Fig. S8a,b ) [14] , [20] . As the reduction of IBM1 transcripts in ibm2 occurred specifically at the 3′ region downstream of the intron containing the heterochromatic domain, we speculated that full-length transcription of IBM1 might be hindered by this sequence. To test that possibility, we generated transgenic plants with an IBM1 construct containing a deletion of this heterochromatic region ( FLAG-His-HA-gIBM1Δi7 ; Fig. 1e ). Indeed, the transgene rescued DNA hypermethylation of IBM1 target genes in the ibm2 mutant ( Fig. 1f , Supplementary Fig. S8c ), demonstrating that phenotypes of ibm2 mutants were mediated by reduced functional transcript of IBM1 . A control IBM1 construct containing the heterochromatic domain did not rescue the ibm2 phenotype, confirming that this region inhibits the expression of IBM1 when the function of IBM2 is compromised. Heterochromatic introns in the Arabidopsis and rice genomes To further identify the possible IBM2 targets in the Arabidopsis genome, we searched for genes that showed expression changes in response to ibm2 mutation, by analysing mRNA-seq data. The most interesting features of the seventh intron of IBM1 are that it is relatively long compared with the remainder of the Arabidopsis genome and it includes the aforementioned heterochromatic domain. Compared to other well-studied plant species, the intron size in Arabidopsis is generally shorter [8] , [21] . Still, we were able to identify 133 introns that are longer than the seventh intron of IBM1 (1,975 bp). Some of the genes with long introns showed drastic changes in expression patterns in the ibm2 mutant ( Supplementary Data 1 ). Notably, expression changes strongly correlate with the state of DNA methylation of the intron; genes responding to the ibm2 mutation contain long introns associated with DNA methylation at CHG sites ( Fig. 2a , Supplementary Data 1 ). The number of such long heterochromatic introns is low in the genome of Arabidopsis thaliana , but even the rice genome, which is reasonably compact, has a large number of long introns ( Fig. 2b ), and surprisingly, many of them have features of heterochromatin ( Fig. 2c ). We further investigated 79 of the 133 long introns in the Arabidopsis genome, listed in Supplementary Data 1 , and found that 24 introns have insertions of 66 TEs (ref. [22] 22). Interestingly, introns with CHG hypermethylation tend to have TE insertions ( Supplementary Data 1 ), indicating that intragenic TEs are the major target of the heterochromatic modifications. The majority of inserted TEs are Class II TEs, such as Helitron (38/66 insertions) and MuDR (18/66), while Class I TEs are relatively uncommon (LTR: 6/66, LINE: 1/66). Introns that significantly affect gene expression in ibm2 ( Supplementary Data 1 ) contain 19 TEs that have an average length of 1,068.4 bp, which is twice as long as the average of the remaining 46 TEs (453.4 bp). 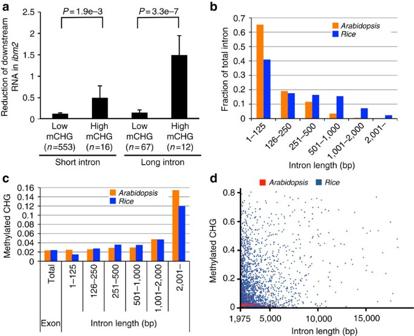Figure 2: Heterochromatic introns in the genomes ofArabidopsisand rice. (a) Expression changes of genes with hypomethylated (Low mCHG) or hypermethylated (High mCHG) short introns (1,975 bp>intron length>1,000 bp), or genes with Low mCHG or High mCHG long introns (intron length≥1,975 bp). ‘High mCHG’ and ‘Low mCHG’ are those with methylation level at CHG sites higher or lower than 0.2.Yaxis: An index representing changes in the 5′/3′ mRNA ratio of the long intron-enclosing genes in response to theibm2mutation. Details are described in Methods.P-values were generated by two-tailedt-tests. (b) The rice genome contains much more abundant long introns than theArabidopsisgenome. (c) Proportion of methylated cytosine at CHG sites compared among introns of different length. The value was derived from sum of mapped cytosines in each class. Long introns tend to have more CHG methylation in bothArabidopsisand rice. (d) The rice genome contains many more long heterochromatic introns than theArabidopsisgenome. Introns longer than the seventh intron ofIBM1(≥1,975 bp) are plotted with the proportion of methylated C in CHG sites, a hallmark of heterochromatin. Red and blue dots represent introns ofArabidopsisand rice, respectively. Overall, 352 of 3,708 long introns of rice and 28 of 133 long introns ofArabidopsisare not plotted, because of inefficient mapping by reads of bisulphite-treated DNA (number of counted C<0.5 × intron length). Figure 2: Heterochromatic introns in the genomes of Arabidopsis and rice. ( a ) Expression changes of genes with hypomethylated (Low mCHG) or hypermethylated (High mCHG) short introns (1,975 bp>intron length>1,000 bp), or genes with Low mCHG or High mCHG long introns (intron length≥1,975 bp). ‘High mCHG’ and ‘Low mCHG’ are those with methylation level at CHG sites higher or lower than 0.2. Y axis: An index representing changes in the 5′/3′ mRNA ratio of the long intron-enclosing genes in response to the ibm2 mutation. Details are described in Methods. P -values were generated by two-tailed t -tests. ( b ) The rice genome contains much more abundant long introns than the Arabidopsis genome. ( c ) Proportion of methylated cytosine at CHG sites compared among introns of different length. The value was derived from sum of mapped cytosines in each class. Long introns tend to have more CHG methylation in both Arabidopsis and rice. ( d ) The rice genome contains many more long heterochromatic introns than the Arabidopsis genome. Introns longer than the seventh intron of IBM1 (≥1,975 bp) are plotted with the proportion of methylated C in CHG sites, a hallmark of heterochromatin. Red and blue dots represent introns of Arabidopsis and rice, respectively. Overall, 352 of 3,708 long introns of rice and 28 of 133 long introns of Arabidopsis are not plotted, because of inefficient mapping by reads of bisulphite-treated DNA (number of counted C<0.5 × intron length). Full size image IBM2 promotes RNA processing over intragenic heterochromatin In the Arabidopsis ibm2 mutant, amounts of full-length transcripts spanning heterochromatic introns formed by insertion of TEs were significantly reduced ( Fig. 3a–d , Supplementary Figs. S9 and S10a , Supplementary Data1 , Supplementary Table S2 ). We tested whether long, heterochromatic TEs in introns are, in fact, responsible for transcription defects of these genes in ibm2 , using natural variant alleles without TE insertions. Another natural strain, Landsberg erecta (L er ), does not contain TE insertions in two of these genes ( Fig. 3e ). In these alleles lacking TEs, the ibm2 mutation did not affect the level of full-length transcripts ( Fig. 3f ), indicating that, as in the IBM1 locus, intragenic heterochromatin within these active genes is the target of IBM2 activity. 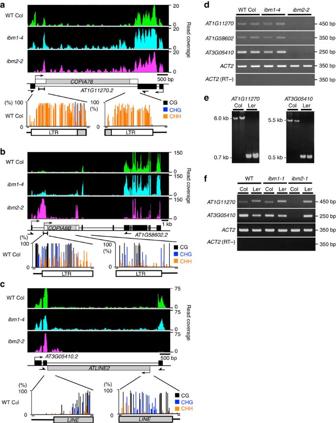Figure 3: IBM2 facilitates transcription of genes with intragenic heterochromatin. (a–c) mRNA read coverage, gene structure and bisulphite analysis of genes with intragenic TEs. Exons of genes and TEs are identified by black and grey boxes, respectively. White boxes represent long terminal repeats (LTRs) of the TEs. Multiple hits of reads on TE sequences, including the LTR, are reflected in the figures. Although 13 intragenic TEs are identified inAT1G58602, only the longest intragenic TE (AT1TE71775/ATCOPIA8B) is shown inb. (d) RT–PCR of TE-enclosing genes with specific primers that are indicated ina–cby arrows. (e) PCR amplification of genomic DNA from wild-type Col and Landsbergerecta(Ler) using primers as ind. (f) RT–PCR of TE-enclosing genes in the indicated genotypes with either Col or Ler background. Figure 3: IBM2 facilitates transcription of genes with intragenic heterochromatin. ( a – c ) mRNA read coverage, gene structure and bisulphite analysis of genes with intragenic TEs. Exons of genes and TEs are identified by black and grey boxes, respectively. White boxes represent long terminal repeats (LTRs) of the TEs. Multiple hits of reads on TE sequences, including the LTR, are reflected in the figures. Although 13 intragenic TEs are identified in AT1G58602 , only the longest intragenic TE ( AT1TE71775 / ATCOPIA8B ) is shown in b . ( d ) RT–PCR of TE-enclosing genes with specific primers that are indicated in a – c by arrows. ( e ) PCR amplification of genomic DNA from wild-type Col and Landsberg erecta (L er ) using primers as in d . ( f ) RT–PCR of TE-enclosing genes in the indicated genotypes with either Col or Ler background. Full size image In general, the presence of TEs in a gene unit often results in transcription elongation defects [9] . However, we found that in wild-type Col, the majority of mature poly(A) mRNAs spanned heterochromatic regions ( Fig. 4 , Supplementary Fig. S9 ), suggesting that the transcription machinery can produce read-through transcripts of intragenic TEs without disturbing the repressive epigenetic marks ( Fig. 3a–d , Supplementary Fig. S9 ). In the ibm2 mutant, however, transcripts spanning the intragenic heterochromatin were drastically reduced, and instead, proportions of shorter forms of transcript variants were increased ( Fig. 4 , Supplementary Data 1 ). Changes in 3′ processing patterns of these genes in the ibm2 mutant suggest that IBM2 might facilitate passage of transcription machinery through the heterochromatic domain marked by repressive epigenetic modifications. Alternatively, IBM2 might have a post-transcriptional function for RNA processing. To test these possibilities, we analysed RNA polymerase II (Pol II) density at the IBM1 locus and TE-enclosing genes by chromatin immunoprecipitation (ChIP)-quantitative PCR. Importantly, loss of IBM2 function did not abolish localization of Pol II at regions downstream of intragenic heterochromatin ( Fig. 5a–d , Supplementary Fig. S10b,c ), suggesting that IBM2 does not affect passage of transcription machinery, but rather is involved in post-transcriptional RNA processing ( Fig. 5f ). IBM2 has an RRM, which is found in proteins functioning in the 3′ end processing of mRNAs, such as FPA and FCA in Arabidopsis [23] , [24] . fpa and fca mutants induce an extensive transcriptional read-through of the 3′ region of genes [25] , [26] . Although the functions of IBM2 and FCA / FPA in 3′ processing may have a mechanistic overlap, ibm2 mutation rather induces premature termination around heterochromatic domains. 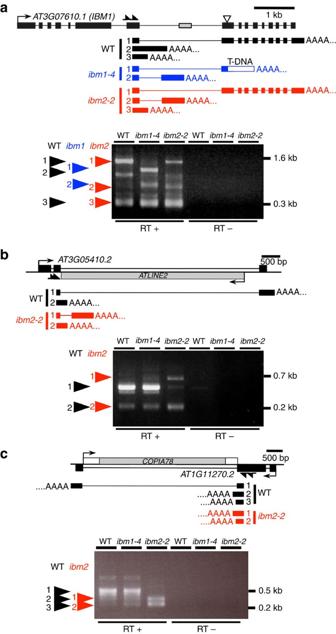Figure 4: 3′ Rapid Amplification of cDNA Ends (RACE) ofIBM1and a gene with an intragenic TE. (a) 3′ RACE ofIBM. Upper panel: Structure of theIBM1locus and polyadenylated mRNA variants detected by 3′ RACE. Exons and spliced introns confirmed by sequencing analysis are shown as black/red boxes and lines, respectively. Primers used for 3′ RACE are indicated by arrows. The T-DNA insertion site of theibm1-4allele is indicated by a white triangle. The white box in transcript 1 inibm1-4indicates fusion of the DNA sequence derived from the T-DNA to theIBM1transcript. Lower panel: Gel picture of DNA fragments amplified by 3′ RACE. DNA fragments indicated by arrowheads were cloned and sequenced, and the representative clones were shown in the upper panel. (b) 3′ RACE of a TE-enclosing geneAT3G05410shown asa. (c) 3′ RACE of a TE-enclosing geneAT1G11270shown asa. Figure 4: 3′ Rapid Amplification of cDNA Ends (RACE) of IBM1 and a gene with an intragenic TE. ( a ) 3′ RACE of IBM . Upper panel: Structure of the IBM1 locus and polyadenylated mRNA variants detected by 3′ RACE. Exons and spliced introns confirmed by sequencing analysis are shown as black/red boxes and lines, respectively. Primers used for 3′ RACE are indicated by arrows. The T-DNA insertion site of the ibm1-4 allele is indicated by a white triangle. The white box in transcript 1 in ibm1-4 indicates fusion of the DNA sequence derived from the T-DNA to the IBM1 transcript. Lower panel: Gel picture of DNA fragments amplified by 3′ RACE. DNA fragments indicated by arrowheads were cloned and sequenced, and the representative clones were shown in the upper panel. ( b ) 3′ RACE of a TE-enclosing gene AT3G05410 shown as a . ( c ) 3′ RACE of a TE-enclosing gene AT1G11270 shown as a . 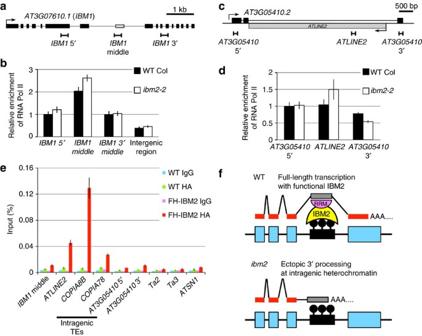Figure 5: Pol II and IBM2 densities atIBM1and intragenic heterochromatin. (a) Structure of theIBM1locus. (b) ChIP-qPCR analysis for Pol II at theIBM1locus. Target regions are indicated in (a). Data were from two independent biological replications for each genotype, normalized by the Pol II signal atACT7. Bars represent means of six independent IPs±s.d. (n=6). The value atIBM15′ in WT Col was set as 1. (c) Structure of the TE-enclosing geneAT3G05410. (d) Chromatin immunoprecipitation (ChIP)-quantitative PCR (ChIP-qPCR) analysis for Pol II atAT3G05410performed as in (b). (e) ChIP-qPCR analysis for FLAG–HA–IBM2 (FH–IBM2) at intragenic TEs with anti-HA antibody (HA) or control immunoglobulin G (IgG). Target regions of intragenic TEs are indicated in (a,c) andFig. 3a. Experiments were performed twice with independently fixed samples, and a representative experiment was shown. Bars represent means of three independent IPs±s.d. (WT HA, FH–IBM2 HA:n=3), or means of two independent control IPs (WT IgG, FH–IBM2 IgG:n=2). The IBM2 signal for the heterochromatic domain in theIBM1locus tended to be weaker than those of other IBM2 targets, possibly because the heterochromatin region is shorter. (f) A model summarizing the function of IBM2, which facilitates appropriate processing of the transcripts (red lines) over intragenic heterochromatin (black box and lollipops). Light-blue boxes represent exons. The grey box in the primary transcript represents the sequence corresponding to the heterochromatic region. RRM, RNA recognition motif. Full size image Figure 5: Pol II and IBM2 densities at IBM1 and intragenic heterochromatin. ( a ) Structure of the IBM1 locus. ( b ) ChIP-qPCR analysis for Pol II at the IBM1 locus. Target regions are indicated in ( a ). Data were from two independent biological replications for each genotype, normalized by the Pol II signal at ACT7 . Bars represent means of six independent IPs±s.d. ( n =6). The value at IBM1 5′ in WT Col was set as 1. ( c ) Structure of the TE-enclosing gene AT3G05410 . ( d ) Chromatin immunoprecipitation (ChIP)-quantitative PCR (ChIP-qPCR) analysis for Pol II at AT3G05410 performed as in ( b ). ( e ) ChIP-qPCR analysis for FLAG–HA–IBM2 (FH–IBM2) at intragenic TEs with anti-HA antibody (HA) or control immunoglobulin G (IgG). Target regions of intragenic TEs are indicated in ( a , c ) and Fig. 3a . Experiments were performed twice with independently fixed samples, and a representative experiment was shown. Bars represent means of three independent IPs±s.d. (WT HA, FH–IBM2 HA: n =3), or means of two independent control IPs (WT IgG, FH–IBM2 IgG: n =2). The IBM2 signal for the heterochromatic domain in the IBM1 locus tended to be weaker than those of other IBM2 targets, possibly because the heterochromatin region is shorter. ( f ) A model summarizing the function of IBM2, which facilitates appropriate processing of the transcripts (red lines) over intragenic heterochromatin (black box and lollipops). Light-blue boxes represent exons. The grey box in the primary transcript represents the sequence corresponding to the heterochromatic region. RRM, RNA recognition motif. Full size image In addition to RRM, IBM2 has a BAH domain, which is often found in proteins associated with chromatin [27] , [28] , [29] . As intragenic heterochromatin seems to be a general target of IBM2 ( Fig. 2a ), we tested whether IBM2 is localized at TEs. For that purpose, we generated transgenic lines that express IBM2 protein fused with FLAG and haemagglutinin (HA) epitopes ( Supplementary Fig. S11a,b ). ChIP-quantitative PCR experiments with anti-HA antibody demonstrated that IBM2 protein was indeed enriched at intragenic TEs ( Fig. 5e ). Intriguingly, however, the signal was much weaker in TEs outside transcription units, suggesting that intragenic heterochromatin has a unique property that recruits IBM2 when combined with canonical heterochromatic epigenetic modifications. In this study, we identified a novel cellular mechanism that promotes production of full-length mRNAs over intragenic heterochromatin ( Fig. 5f ). The mechanism involving IBM2, which allows the presence of long TE sequences within transcription units, should be important especially in higher eukaryotic species with many more heterochromatic TEs in the genome [1] , [30] . In addition, considering that the heterochromatic domain in the IBM1 is associated with an organelle genome sequence, there may be additional targets for IBM2 besides intragenic TEs ( Supplementary Data 1 ). Maintenance of heterochromatic epigenetic states at the domains seems to be important for full-length transcription of the genes including IBM1 , as erasure of heterochromatic epigenetic modifications results in a reduction of full-length transcripts of genes with heterochromatic domains, as observed in ibm2 (refs 14 , 20 , 31 ). However, ibm2 mutation affects expression of IBM1 without changing DNA methylation at the intron ( Supplementary Fig. S8a,b ). Therefore, IBM2 may act downstream of repressive epigenetic modifications by binding to the heterochromatic domain or to proteins required for transcriptional repression, via its BAH domain ( Fig. 5e ) [27] , [28] , [29] . Notably, IBM2 is recruited more efficiently to intragenic heterochromatin than to heterochromatin outside genes ( Fig. 5e ). On the other hand, IBM2 is not directly associated with transcription machinery ( Supplementary Fig. S11c ). These results suggest that epigenetic marks or proteins other than those in canonical heterochromatin may be involved in recruiting IBM2 to targeted loci. Our results demonstrate that the transcription machinery passes over intragenic TEs without changing the epigenetic marks of silent chromatin ( Fig. 3a–c , Supplementary Fig. S9 ). That was surprising to us, because transcription elongation is generally associated with recruitment of chromatin-modifying enzymes, resulting in accumulation of active chromatin marks such as histone H3K4 methylation and H3K36 methylation [3] , [4] , [5] . In budding yeast, for example, transcription elongation through heterochromatic domains resulted in displacement of silencing proteins and loss of heterochromatic structure [32] . On the other hand, establishment of heterochromatin at pericentromeric repeats in fission yeast requires a Pol II read-through of the regions, in which Pol II transcripts recruit RNAi complex and histone H3K9 methylase [33] , [34] . Similarly, it has been reported that Pol II-dependent transcription in Arabidopsis in an intergenic region can induce small interfering RNA-directed gene silencing [35] , [36] . In the case of the PAI locus in Arabidopsis , H3K9 methylation and DNA methylation are maintained despite read-through transcription of the locus, which depend on small RNAs produced by Dicers [37] . Therefore, it would be interesting to know if Pol II transcripts generated from intragenic TEs reinforce heterochromatic structures by recruiting RNA-directed DNA methylation machinery [12] . Mechanisms that trigger premature transcriptional termination around the intragenic heterochromatin in ibm2 are presently unknown. In mammals, insertion of intragenic IAP elevates usage of cryptic poly(A) signals present in gene units, which could be due to ectopic transcription of antisense transcripts from internal promoters of TE [10] , [11] . Therefore, it is possible that IBM2 prevents premature transcriptional termination by suppressing antisense transcription from cryptic promoters. Indeed, the production of antisense transcripts was detected from the heterochromatic domain of the IBM1 locus [20] . Alternatively, binding of the RRM domain to pre-mRNA might directly suppress utilization of alternative poly(A) signals near or within heterochromatic domain, which would eventually promote splicing of the intron containing heterochromatin [38] . During evolution, or in response to perturbations of the environment, heterochromatic elements might manifest themselves via the changes in epigenetic states [39] . It has been demonstrated that full-length IBM1 mRNA is reduced in the met1 mutant, due to a loss of DNA methylation at the heterochromatinc domain [20] , [40] . Because IBM1 encodes a histone H3K9 demethylase [19] , the heterochromatic domain in IBM1 may function as a genome-wide fine-tuning mechanism, balancing active and repressive states of genes and TEs, through the control of full-length transcription of IBM1 [20] . Interestingly, the organelle-like sequence is also present in the Arabidopsis lyrata orthologue of IBM1 ( Supplementary Fig. S12 ), suggesting that its insertion originated before the separation of these species. Moreover, one of the targets of IBM2 is a recently identified TE family that becomes mobile when plants are exposed to heat stress ( Fig. 3a ) [41] , [42] . Thus, mechanisms to cope with heterochromatin allow the evolution of complex gene controls in higher eukaryotes, and could be the origin of diverse epigenetic phenomena [43] , [44] , [45] , [46] , [47] , [48] , [49] . IBM2 genes are conserved in other plant species ( Supplementary Fig. S13 ), and the BAH and RRM domains are evolutionarily conserved motifs in eukaryotes. It will be interesting to learn the significance of this pathway in other species possessing more intragenic TEs. Screening and isolation of the Arabidopsis ibm2-1 mutant Screening of ibm mutants was performed with an ethyl methanesulfonate (EMS)-mutagenized Arabidopsis population [17] . A Col line containing the ibm2-1 allele was crossed to a wild-type L er strain, and ~200 F2 plants and F3 descendants were used for fine mapping. The ibm2-1 mutation was mapped to the top arm of chromosome 5, at an interval of ~330 kb between the polymorphisms PERL0881671 and PERL0884446. Candidate genes were sequenced, and we found that the gene, AT5G11470 , has a single-base deletion of G, 1,603-bp downstream from the ATG translation start site, which results in a frameshift and creation of a TGA translation stop codon 39 bp downstream. The ibm2-1 mutation was complemented by a 6.6-kb genomic DNA fragment containing the AT5G11470 gene (see below), confirming that the gene is identical to IBM2 . ibm2-1 and wild-type IBM2 alleles were distinguished by digestability of the PCR product by Eco RV, using the primers IBM2-CAPs P1 and IBM2-CAPs P2. PCR primers used in this study are listed in Supplementary Table S3 . Plant growth conditions and plant strains Plants were grown under long-day conditions (16 h, light; 8 h, dark) at 22 °C. ddm1-1 , cmt3-i11, kyp, ibm1-1 and ibm1-4 mutations have been reported [17] , [50] , [51] , [52] . ibm2-2 (GABI-Kat: 045A07: NASC Code N404231) and ibm2-3 (GABI-Kat: 484B11) were obtained from NASC [52] or GABI-Kat [53] , respectively. Heterozygous ibm2-2 and ibm2-3 plants were backcrossed at least once to wild-type Col and used after confirming segregation of additional T-DNAs by Southern analysis. The ibm2-1 mutant was used after backcrossing either to wild-type Col or to wild-type L er more than six times. DNA methylation analysis For PCR-based DNA methylation analysis [54] , 200 ng of genomic DNA was digested with Bgl II and EcoR I, in a 20-μl reaction mix. Control ‘undigested’ sample was digested with EcoR I alone. After digestion, PCR was performed using 1 μl of digested sample as a template. For bisulphite sequencing analysis [55] , 0.25–1 μg of heat-denatured genomic DNA in 20 μl H 2 O was incubated with 1/9 vol of 3 M NaOH for 20 min at 37 °C. Next, 275 μl of 10 M bisulphite solution was added to the denatured DNA sample and incubated at 70 °C for 1 h. Bisulphite-treated DNA was purified and desulphonated using an EZ DNA Methylation Kit (Zymo Research) according to the manufacturer’s instructions, and eluted with 20 μl of elution buffer. PCR used 2 μl of DNA as a template. A total of 16–20 clones were sequenced for each region. Genome-wide DNA methylation analysis To estimate genome-wide DNA methylation levels in introns, sequence data were downloaded from GEO (accession GSE10966 for Arabidopsis Col-0 (ref. 14 ) and GSE22591 for rice shoot [56] ). Reads were mapped to reference genomes (Release 10 of the Arabidopsis Information Resources; Release 7 of the MSU Rice Genome Annotation Project) using the Bowtie alignment algorithm [57] under conditions described [58] . Only uniquely mapped reads were used for the analysis. Reverse transcription–PCR Total RNA of wild-type and mutant plants was isolated from Arabidopsis leaves or flowers, using RNAiso (Takara) according to the manufacturer’s instructions. RNA was further treated with DNaseI (Takara) followed by phenol/chloroform extraction and ethanol precipitation. cDNA was synthesized using a TAKARA RNA PCR kit (AMV) Ver.3.0 (Takara) with oligo-(dT) primer. A total of 1 μg RNA in the reverse transcription (RT) reaction mixture (total 20 μl) was reverse transcribed at 42–50 °C for 1 h, followed by heat inactivation at 95 °C for 5 min. 1 μl of the RT reaction was used as a template for PCR (total 20 μl) [54] . 3′ Rapid Amplification of cDNA Ends was performed using oligo-dT primers followed by the first round of PCR using gene-specific primers and the first oligo-dT-specific primer ( Supplementary Table S3 ). Amplified fragments were diluted and further used for the second round of PCR using another gene-specific primer and a second oligo-dT-specific primer ( Supplementary Table S3 ). Quantitative RT–PCR (qRT-PCR) was performed using SYBR Premix Ex Taq (Takara). mRNA-seq analysis Total RNA of wild-type Col, ibm1-4 and ibm2-2 plants homozygous for three generations (F4) was isolated from unopened flower buds using RNAiso (Takara), followed by a cleanup using an RNAeasy Minikit (Qiagen). RNA samples were sent to Hokkaido System Science (Hokkaido, Japan), treated with the mRNA-seq sample prep kit (Illumina), and sequenced by illumina GAII. mRNA-seq data (75-base reads) were aligned to the Arabidopsis genome (TAIR10) using Tophat 1.0.14.OSX (ref. 59 ). Read coverage of gene models was visualized using Integrated Genome Browser 6.5 (ref. 60 ) and CLC Bio Genomics Workbench software (CLC bio). Estimating effects of ibm2 on transcripts over introns Transcript reads were counted before and after respective introns. The effect of the ibm2 mutation is shown by –log e (((observed post-intron read number in ibm2 )+1)/(expected post-intron read number in ibm2 )+1). The expected post-intron read number in ibm2 is calculated by (pre-intron read number in ibm2 ) × (post-intron read number in wild type)/(pre-intron read number in wild type). If at least one of these three parameters was 0, then that intron was not included in the analysis. For long introns, At1g24880.1 and At1g25054.1 were not included because the methylation level could not be examined, most likely due to inefficient mapping of the repeats. Reads for At1g11270.2 were not mapped, but At1g11270.2 was included in the ‘High mCHG’ class, because of its high non-CG methylation ( Fig. 3a ). Generation of transgenic plants A genomic DNA fragment including AT5G11470 was designed to express a protein fused with 2xFLAG and 2xHA epitopes to the N terminus of IBM2 by the endogenous promoter ( FLAG–HA–gIBM2 ), cloned into the pRI909 vector (Takara) and transformed into ibm2-1 heterozygous plants. Complementation of the ibm2-1 mutation was confirmed by the absence of DNA methylation in T2–T4 ibm2 homozygous plants at several loci, including the BNS locus, using DNA methylation PCR ( Supplementary Fig. S11a ). The presence of FLAG–HA–IBM2 protein in the nuclear extract of transgenic plants was confirmed by western blotting with an anti-HA antibody (Roche; 2013819) ( Supplementary Fig. S11b ). For complementation of ibm2-2 with IBM1 , a 7.8-kb piece of the genomic IBM1 DNA fragment was designed to express a protein fused with FLAG, 6xHis and HA epitopes to the N-terminal of IBM1 with the endogenous IBM1 promoter ( FLAG–His–HA–gIBM1 ) ( Fig. 1e ). The FLAG–His–HA–gIBM1 was able to rescue ibm1 phenotypes. In addition, a FLAG–His–HA–gIBM1 transgene with a 720-bp deletion of the sequence similar to the organelle genome in the seventh intron was constructed ( FLAG–His–HA–gIBM1Δi7 ) ( Fig. 1e ). These transgenes were cloned into pRI909 vector and transformed into ibm2-2 heterozygous plants. Immunoprecipitation and ChIP assay Nuclei of wild-type Col and FLAG–HA–gIBM2 transgenic plants were isolated using a CelLyticTM PN Isolation/Extraction kit (Sigma-Aldrich) according to the manufacturer’s instructions. Nuclei were suspended in buffer A (10 mM HEPES (pH 7.9)/1.5 mM MgCl 2 /10 mM KCl/0.5 mM dithiothreitol/0.1 mM phenylmethylsulphonyl fluoride). After centrifugation, nuclei were suspended in buffer C (20 mM HEPES (pH 7.9)/25% (v/v) glycerol/0.42 M NaCl/1.5 mM MgCl 2 /0.2 mM EDTA/0.5 mM dithiothreitol/0.1 mM phenylmethylsulphonyl fluoride) with vortexing for 40 min. After centrifugation, supernatant was used as the nuclear extract for further experiments. For the Pol II pull-down assay, nuclear extract from FLAG–HA–gIBM2 transgenic plants was incubated with either 2 μg of anti-Pol II antibody (Abcam, ab817) or 20 μl of anti-HA affinity matrix (Roche, 1815016). Anti-Pol II antibody complex was further precipitated with 20 μl of Dynabeads M-280 anti-mouse IgG (Invitrogen, 112-01D). Beads were washed and boiled for 10 min in SDS loading buffer, and proteins were subjected to SDS–PAGE, followed by western blotting. Pol II protein and IBM2 protein fused with HA tag were detected with anti-Pol II antibody (Abcam, ab817; 1:500 dilution) and anti-HA antibody (Roche, 2013819; 1:500 dilution), respectively. The ChIP assay was essentially performed as described [17] , with minor modifications. Briefly, 3 g of leaves were fixed with fixation buffer (10 mM Tris-HCl, pH 7.5, 0.1 M sucrose, 1% formaldehyde). Nuclei of wild-type Col and ibm2 plants were isolated using a CelLyticTM PN Isolation/Extraction kit (Sigma-Aldrich) according to the manufacturer’s instructions, and were lysed and sonicated. Chromatin was immunoprecipitated by overnight incubation with 2 μg of anti-Pol II antibody (Abcam, ab817) bound to Dynabeads M-280 anti-mouse IgG (Invitrogen, 112-01D). Purified DNA was analysed by quantitative RT–PCR, using SYBR Premix Ex Taq (Takara). For precipitation of chromatin bound with FLAG–HA–IBM2, nuclei of wild-type Col and ibm2-1 plants complimented with FLAG–HA–gIBM2 were isolated as described above. Sonicated chromatin was precleared with Rat-IgG (Abcam, ab37361) and protein G magnetic beads (Invitrogen, 100-03D), and 2 μg of anti-HA antibody (Roche, 2013819) or 2 μg of control IgG were added for overnight incubation. Antibody complexes were precipitated with protein G magnetic beads and washed. Purified DNA was analysed by quantitative RT–PCR as described above. Accession code: Sequencing data have been deposited in the DDBJ Sequence Read Archive under accession code DRP001015 . How to cite this article: Saze, H. et al . Mechanism for full-length RNA processing of Arabidopsis genes containing intragenic heterochromatin. Nat. Commun. 4:2301 doi: 10.1038/ncomms3301 (2013)